Discovery of acetylene hydratase activity of the iron–sulphur protein IspH The final step of the methylerythritol phosphate isoprenoid biosynthesis pathway is catalysed by the iron–sulphur enzyme IspH, producing the universal precursors of terpenes: isopentenyl diphosphate and dimethylallyl diphosphate. Here we report an unforeseen reaction discovered during the investigation of the interaction of IspH with acetylene inhibitors by X-ray crystallography, Mößbauer, and nuclear magnetic resonance spectroscopy. In addition to its role as a 2H + /2e − reductase, IspH can hydrate acetylenes to aldehydes and ketones via anti-Markovnikov/Markovnikov addition. The reactions only occur with the oxidised protein and proceed via η 1 -O-enolate intermediates. One of these is characterized crystallographically and contains a C4 ligand oxygen bound to the unique, fourth iron in the 4Fe-4S cluster: this intermediate subsequently hydrolyzes to produce an aldehyde product. This unexpected side to IspH reactivity is of interest in the context of the mechanism of action of other acetylene hydratases, as well as in the design of antiinfectives targeting IspH. Metalloproteins containing [Fe 4 S 4 ] clusters carry out a broad series of reactions [1] , [2] . For example, aconitase [3] catalyses the hydration of the alkene-containing species cis -aconitate to citrate and iso-citrate, whereas ferredoxins [1] , [4] mediate electron transfer reactions. In isoprenoid biosynthesis, the protein ( E )-4-hydroxy-3-methyl-but-2-enyl diphosphate (HMBPP, 1 ) reductase (IspH, Fig. 1a ) performs a 2H + /2e − reduction and deoxygenation of 1 , yielding isopentenyl diphosphate ( 2 ) and dimethylallyl diphosphate ( 3 ) ( Fig. 1b ) [5] , [6] , [7] , [8] , [9] , [10] , [11] , [12] . This reaction is of interest in the context of drug development, as IspH is essential for the growth of many pathogenic bacteria, as well as of malaria parasites [13] , [14] , [15] . 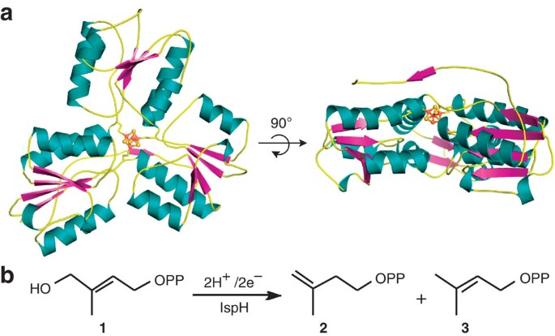Figure 1: Structure and enzymatic activity of IspH. (a) Top and side view of the overall crystal structure of IspH protein fromEscherichia coli. The protein comprises three structurally similar domains with a [Fe4S4] cluster in the active site. The cluster is displayed as ball and stick model, whereas the protein is shown as cartoon. (b) Reaction of (E)-4-hydroxy-3-methylbut-2-enyl diphosphate (1) to isopentenyl diphosphate (2) and dimethylallyl diphosphate (3) catalysed by the 2H+/2e−reductase IspH. This conversion represents the final step in the non-mevalonate pathway leading to the universal precursors,2and3, in isoprenoid biosynthesis. Figure 1: Structure and enzymatic activity of IspH. ( a ) Top and side view of the overall crystal structure of IspH protein from Escherichia coli . The protein comprises three structurally similar domains with a [Fe 4 S 4 ] cluster in the active site. The cluster is displayed as ball and stick model, whereas the protein is shown as cartoon. ( b ) Reaction of ( E )-4-hydroxy-3-methylbut-2-enyl diphosphate ( 1 ) to isopentenyl diphosphate ( 2 ) and dimethylallyl diphosphate ( 3 ) catalysed by the 2H + /2e − reductase IspH. This conversion represents the final step in the non-mevalonate pathway leading to the universal precursors, 2 and 3 , in isoprenoid biosynthesis. Full size image Here we report that, in addition to its role as a 2H + /2e − reductase in isoprenoid biosynthesis, IspH can catalyse a second class of reactions: the addition of water to acetylene groups to produce aldehyde and ketone products. These reactions are shown to occur via η 1 -O-enolate intermediates, one of which is characterized by crystallography, with the ligand's oxygen at C4 being found to bind to the unique fourth iron of the [Fe 4 S 4 ] cluster. This acetylene hydration is equivalent to the reaction catalysed by the W(IV)-containing protein acetylene hydratase [16] , where enolate formation has recently been proposed on theoretical grounds to be part of the mechanism [17] . Mößbauer studies of acetylene inhibitors We started with a Mößbauer spectroscopic investigation of the IspH inhibitors [18] propynyl diphosphate ( 4 ), but-3-ynyl diphosphate ( 5 ), and pent-4-ynyl diphosphate ( 6 ) bound to oxidised IspH from E. coli ( Fig. 2 ). All compounds gave similar Mößbauer spectra ( Fig. 3a–c ) with quadrupole splittings (ΔE Q ) of ~1.1 mm s −1 and isomer shifts (δ Fe ) of ~0.45 mm s −1 . These values differ from those seen in ligand-free IspH ( Fig. 3d ) [19] . However, they are similar to those observed on addition of the HMBPP substrate ( 1 ) to the enzyme, where the quadrupole splitting of the fourth Fe changes from 1.91 to 1.00 mm s −1 , and the isomer shifts decrease from 0.89 to 0.53 mm s −1 [19] . As noted by Seemann et al ., based on previous work with aconitase and model systems, this indicates conversion from a 3S,3N/O (octahedral) to a 3S,1O (tetrahedral) coordination sphere of the iron [19] , [20] . The Mößbauer results of IspH in complex with 4 - 6 also suggest a 3S,1O coordination on inhibitor binding, as reported for the substrate 1 . 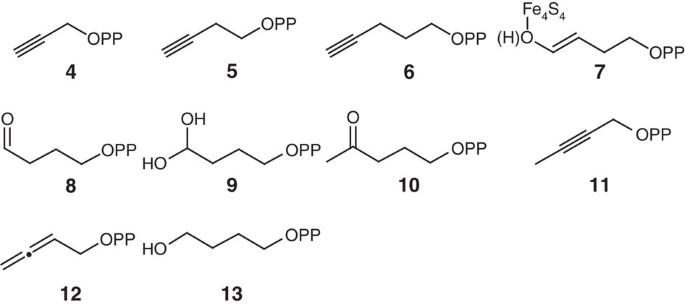Figure 2: Chemical structures of ligands binding to the active site of IspH. The acetylene diphosphates4–6were crystallized in complex with IspH; the hydration products7–10have been observed in crystal structures or by NMR spectroscopy; compounds11–13bind to the catalytic centre of IspH, but are not converted by the enzyme. Figure 2: Chemical structures of ligands binding to the active site of IspH. The acetylene diphosphates 4–6 were crystallized in complex with IspH; the hydration products 7–10 have been observed in crystal structures or by NMR spectroscopy; compounds 11–13 bind to the catalytic centre of IspH, but are not converted by the enzyme. 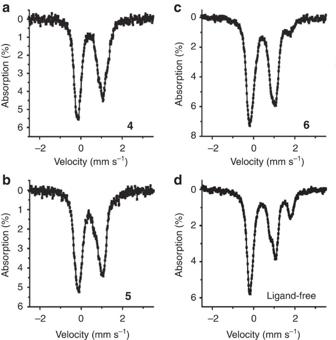Figure 3:57Fe Mößbauer data on IspH–acetylene interactions. Mößbauer spectra of oxidisedE. coliIspH bound to: (a) propynyl diphosphate4(Component 1 (25%)δ=0.52 mm s–1, ΔEQ=1.54 mm s–1; Component 2 (50%)δ=0.45 mm s–1, ΔEQ=1.20 mm s–1; Component 3 (25%)δ=0.41 mm s–1, ΔEQ=0.85 mm s–1); (b) but-3-ynyl diphosphate5(Component 1 (50%)δ=0.45 mm s–1, ΔEQ=1.28 mm s–1; Component 2 (50%)δ=0.39 mm s–1, ΔEQ=0.89 mm s–1); (c) pent-4-ynyl diphosphate6(Component 1 (50%)δ=0.42 mm s–1, ΔEQ=1.54 mm s–1; Component 2 (50%)δ=0.45 mm s–1, ΔEQ=1.20 mm s–1); (d) ligand-free IspH (Component 1 (50%)δ=0.43 mm s–1, ΔEQ=1.28 mm s–1; Component 2 (25%)δ=0.38 mm s–1, ΔEQ=0.86 mm s–1; Component 3 (25%)δ=0.82 mm s–1, ΔEQ=1.98 mm s–1). Full size image Figure 3: 57 Fe Mößbauer data on IspH–acetylene interactions. Mößbauer spectra of oxidised E. coli IspH bound to: ( a ) propynyl diphosphate 4 (Component 1 (25%) δ =0.52 mm s –1 , ΔE Q =1.54 mm s –1 ; Component 2 (50%) δ =0.45 mm s –1 , ΔE Q =1.20 mm s –1 ; Component 3 (25%) δ =0.41 mm s –1 , ΔE Q =0.85 mm s –1 ); ( b ) but-3-ynyl diphosphate 5 (Component 1 (50%) δ =0.45 mm s –1 , ΔE Q =1.28 mm s –1 ; Component 2 (50%) δ =0.39 mm s –1 , ΔE Q =0.89 mm s –1 ); ( c ) pent-4-ynyl diphosphate 6 (Component 1 (50%) δ =0.42 mm s –1 , ΔE Q =1.54 mm s –1 ; Component 2 (50%) δ =0.45 mm s –1 , ΔE Q =1.20 mm s –1 ); ( d ) ligand-free IspH (Component 1 (50%) δ =0.43 mm s –1 , ΔE Q =1.28 mm s –1 ; Component 2 (25%) δ =0.38 mm s –1 , ΔE Q =0.86 mm s –1 ; Component 3 (25%) δ =0.82 mm s –1 , ΔE Q =1.98 mm s –1 ). Full size image Propynyl diphosphate (4) is not converted by IspH Subsequently, we performed co-crystallization of compounds 4–6 bound to oxidised IspH and analysed the ligand-bound X-ray structures obtained. As can be seen with 4 ( Fig. 4a ), the acetylene group is not bonded to the fourth Fe (Fe–C distances of 3.4–3.5 Å), rather, there is a water molecule (or, in principle, a hydroxide ion) bound to the [Fe 4 S 4 ] cluster with a Fe-O bond length of 2.1 Å, essentially the same as in the alkoxide complex formed by oxidised IspH and HMBPP ( 1 ) [21] . The crystal structure of IspH in complex with 4 gives an explanation of the 57 Fe Mößbauer results: the δ Fe and ΔE Q values for 1 as well as 4 bound to IspH are essentially the same because both species contain a [Fe 4 S 4 ] cluster with 3S,1O coordination to the apical Fe. 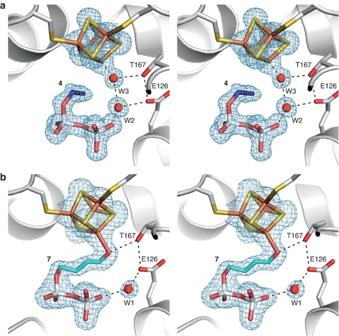Figure 4: Stereo presentation of theE. coliIspH active site with ligands 4 and 7. Ligands, [Fe4S4] clusters and side chains of E126 as well as T167 are displayed as stick models. The protein backbone is presented as coil model (grey) and solvent molecules as spheres (red). A2FO-FComit electron density map (blue mesh, contoured at 1.4 σ) is shown for the [Fe4S4] cluster, the ligand, and the solvent molecules in the first coordination sphere; dotted lines indicate coordination and hydrogen bonds. (a) Crystal structure of IspH bound to propynyl diphosphate (4). The diphosphate group of the ligand binds in the same orientation as observed for the substrate1(ref.21), but no interaction between the alkyne group and the iron–sulphur cluster were observed. Two water molecules are located in the central cavity: W3 coordinates to the fourth site of the apical iron of the [Fe4S4] cluster and W2 is stabilized by E126Oεas well as the diphosphate group. (b) IspH active site with the η1-enolate7and water molecule W1. IspH hydrates but-3-ynyl diphosphate (5) to the corresponding aldehyde8. Figure 4: Stereo presentation of the E. coli IspH active site with ligands 4 and 7. Ligands, [Fe 4 S 4 ] clusters and side chains of E126 as well as T167 are displayed as stick models. The protein backbone is presented as coil model (grey) and solvent molecules as spheres (red). A 2F O -F C omit electron density map (blue mesh, contoured at 1.4 σ) is shown for the [Fe 4 S 4 ] cluster, the ligand, and the solvent molecules in the first coordination sphere; dotted lines indicate coordination and hydrogen bonds. ( a ) Crystal structure of IspH bound to propynyl diphosphate ( 4 ). The diphosphate group of the ligand binds in the same orientation as observed for the substrate 1 (ref. 21 ), but no interaction between the alkyne group and the iron–sulphur cluster were observed. Two water molecules are located in the central cavity: W3 coordinates to the fourth site of the apical iron of the [Fe 4 S 4 ] cluster and W2 is stabilized by E126O ε as well as the diphosphate group. ( b ) IspH active site with the η 1 -enolate 7 and water molecule W1. IspH hydrates but-3-ynyl diphosphate ( 5 ) to the corresponding aldehyde 8 . Full size image IspH converts but-3-ynyl diphosphate (5) to an aldehyde Although the Mößbauer spectroscopic results with 4 and 5 are similar, the X-ray structure of IspH in complex with 5 reveals, surprisingly, an enolate complex ( Fig. 4b ). The diphosphate backbone of 5 binds to the same pocket as found with 1 and 4 ; however, the ligand has undergone a hydration reaction, forming 7 . The crystal structure determined at 2.0 Å resolution clearly indicates formation of an η 1 -O-enolate complex having an Fe–O bond length of 2.0 Å and, as with the IspH-substrate complex [21] , binding of 7 to IspH protects the [Fe 4 S 4 ] cluster from O 2 , with IspH bound to ( E )-4-hydroxybut-3-enyl diphosphate ( 7 ) being remarkably stable under aerobic conditions. Furthermore, this complex actually turns over, forming the aldehyde 4-oxobutyl diphosphate ( 8 ), as evidenced by the appearance of a 1 H NMR peak at 9.72 p.p.m. ( Fig. 5a ). In aqueous solution, such aldehydes exist in part as hydrates (gem-diols), and the J-couplings seen in Fig. 5a are consistent with the presence of both the free aldehyde as well as 4,4-dihydroxybutyl diphosphate ( 9 ), just as reported previously with 3-formyl-1-butyl diphosphate [22] . When 5 is added to IspH in D 2 O, the 1 H NMR resonances from C3 at 2.63 p.p.m. (the aldehyde, 8 ) and 1.65 p.p.m. (the hydrate, 9 ) are absent, because the proton that attaches to C3 in initial enolate formation is now a deuterium, plus, the enolate hydrogen is replaced by a deuterium as well ( Fig. 5b ). These observations are confirmed by electrospray ionisation mass spectrometry (ESI–MS) ( Supplementary Fig. S1 ) with the results showing formation of an m/e=246.9 amu parent ion, due to water addition to 5 . The hydratase activity of IspH with 5 is 2.0 nmol min −1 mg −1 , lower than that of the tungsten iron–sulphur acetylene hydratase (69 μmol min −1 mg −1 ) [23] . 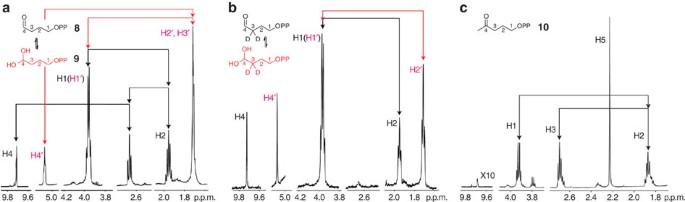Figure 5: NMR spectroscopic characterization of the IspH hydration products. (a)1H NMR spectrum (500 MHz) of aldehyde8(black) and gem-diol9(red) formed on hydration of5by IspH. (b)1H NMR spectrum (500 MHz) showing the products of hydration of5by IspH carried out in D2O, forming [3,3-D2] and [3,3-D2]9. (c)1H NMR spectrum (500 MHz) of the Markovnikov-product10. Figure 5: NMR spectroscopic characterization of the IspH hydration products. ( a ) 1 H NMR spectrum (500 MHz) of aldehyde 8 (black) and gem-diol 9 (red) formed on hydration of 5 by IspH. ( b ) 1 H NMR spectrum (500 MHz) showing the products of hydration of 5 by IspH carried out in D 2 O, forming [3,3-D 2 ] and [3,3-D 2 ] 9 . ( c ) 1 H NMR spectrum (500 MHz) of the Markovnikov-product 10 . Full size image Crystallographic analysis of the IspH:aldehyde (8) complex Structure elucidation of IspH complexed with the aldehyde 8 (prepared by chemical synthesis) at 1.8 Å resolution reveals two ligand conformations: an enolate complex with the apical iron of the [Fe 4 S 4 ] cofactor, and a cyclic conformation of the aldehyde in which its oxygen is able to interact with E126O ε H and the ligand's diphosphate group ( Fig. 6a ). These X-ray structures are consistent with the Mößbauer results, which show that the isomer shift and quadrupole splitting of the fourth iron decrease on ligand binding, as the enolate provides a 3S,1O coordination sphere. 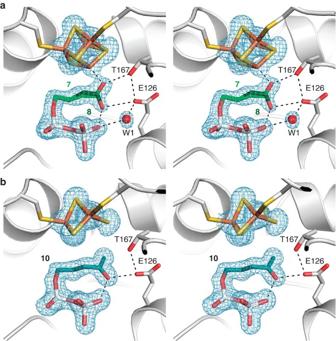Figure 6: Stereo presentation of the central cavity of IspH in complex with ligands 8 and 10. Ligands, cofactors, side chains of E126 as well as T167 are displayed according toFig. 4. A2FO-FComit electron density map (blue mesh, contoured at 1.4 σ) is shown for the [Fe4S4] cluster, the ligand, and the solvent molecules; dotted lines indicate coordination and hydrogen bonds. (a) 4-Oxobutyl diphosphate (8) bound to the IspH active site shows two alternative orientations: a cyclic conformation of the η1-O-enolate7interacting with the fourth iron, and the aldehyde8. The distinct alternative conformations are indicated by the different colours of the carbon atoms. An additional water molecule is located in the W1 position. (b) Structure of IspH in complex with 4-oxopentyl diphosphate (10) displaying an [Fe3S4] cluster. The oxidised IspH catalyzes the Markovnikov addition of a water molecule to pent-4-ynyl diphosphate (6), furnishing10. Figure 6: Stereo presentation of the central cavity of IspH in complex with ligands 8 and 10. Ligands, cofactors, side chains of E126 as well as T167 are displayed according to Fig. 4 . A 2F O -F C omit electron density map (blue mesh, contoured at 1.4 σ) is shown for the [Fe 4 S 4 ] cluster, the ligand, and the solvent molecules; dotted lines indicate coordination and hydrogen bonds. ( a ) 4-Oxobutyl diphosphate ( 8 ) bound to the IspH active site shows two alternative orientations: a cyclic conformation of the η 1 -O-enolate 7 interacting with the fourth iron, and the aldehyde 8 . The distinct alternative conformations are indicated by the different colours of the carbon atoms. An additional water molecule is located in the W1 position. ( b ) Structure of IspH in complex with 4-oxopentyl diphosphate ( 10 ) displaying an [Fe 3 S 4 ] cluster. The oxidised IspH catalyzes the Markovnikov addition of a water molecule to pent-4-ynyl diphosphate ( 6 ), furnishing 10 . Full size image IspH converts pent-4-ynyl diphosphate (6) to a ketone In the case of 6 , the Mößbauer results again indicate a 3S,1O coordination to the apical iron of the [Fe 4 S 4 ] cluster. The crystal structure determined at 1.8 Å resolution ( Fig. 6b ) shows a chemically converted compound inside the IspH active site. However, rather than forming an aldehyde (via anti-Markovnikov addition), the nuclear magnetic resonance (NMR) results ( Fig. 5c ) indicate primarily the formation of 4-oxopentyl diphosphate ( 10 ) via Markovnikov addition, confirming the results of MS ( Supplementary Fig. S1 ). The Mößbauer spectra suggest initial enolate formation as observed with 5 , but surprisingly, the X-ray structure of the complex ( Fig. 6b ) contains a [Fe 3 S 4 ] cluster, so evidently the fourth iron is lost during crystallization. The structure of the ketone 10 is, nevertheless, superimposable with that of the enolate 7 ( Supplementary Fig. S2 , root-mean-square deviation (rmsd)=0.350 Å). The hydratase activity of IspH using 6 as the substrate is 10 nmol min −1 mg −1 , five times higher than that found with 5 . X-ray studies of diphosphates with various functional groups Finally, we investigated the bonding of three additional ligands: 11 – 13 . The methyl-substituted analogue of 4 but-2-ynyl diphosphate ( 11 , Fig. 7a ) as well as buta-2,3-dienyl diphosphate ( 12 , Fig. 7b ) both bind in the active pocket of IspH, although no interaction with the iron–sulphur cluster and no chemical reactions were observed. Interestingly, 4-hydroxybutyl diphosphate ( 13 ) also binds to the oxidised iron–sulphur cluster via O4 with an Fe–O bond length of 2.1 Å ( Fig. 7c ), and adopts a similar conformation to that observed in the alkoxide complex formed by IspH in the presence of 1 ( Supplementary Fig. S3 ). [21] However, 13 did not react further with IspH. 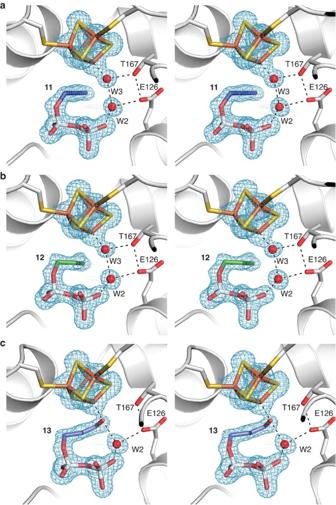Figure 7: Stereo presentation of the active site of IspH in complex with ligands 11, 12 and 13. Protein, cofactors, ligands and solvent molecules are represented according toFig. 4. A2FO-FComit electron density map (blue mesh, 1.4 σ) is shown for the cofactors, the ligands, as well as the water molecules. (a) The IspH:but-2-ynyl diphosphate (11) complex structure displays a [Fe4S4] cluster and an unreacted ligand with two solvent molecules in positions W2 and W3. The alkyne group of11is shifted compared with5, thus there is no interaction with the iron and the carbon chain is rotated towards a hydrophobic pocket formed by A73 and H74. (b) Buta-2,3-dienyl diphosphate (12) adopts a similar orientation and the solvent molecules are located in identical positions as those observed in the structure of IspH bound to11. (c) Binding of 4-hydroxybutyl diphosphate (13) to IspH results in formation of an η1-alkoxide (or possibly, an alcohol) complex with the apical iron of the [Fe4S4] cluster. In addition, one water molecule is evident in the W2 site. Figure 7: Stereo presentation of the active site of IspH in complex with ligands 11, 12 and 13. Protein, cofactors, ligands and solvent molecules are represented according to Fig. 4 . A 2F O -F C omit electron density map (blue mesh, 1.4 σ) is shown for the cofactors, the ligands, as well as the water molecules. ( a ) The IspH:but-2-ynyl diphosphate ( 11 ) complex structure displays a [Fe 4 S 4 ] cluster and an unreacted ligand with two solvent molecules in positions W2 and W3. The alkyne group of 11 is shifted compared with 5 , thus there is no interaction with the iron and the carbon chain is rotated towards a hydrophobic pocket formed by A73 and H74. ( b ) Buta-2,3-dienyl diphosphate ( 12 ) adopts a similar orientation and the solvent molecules are located in identical positions as those observed in the structure of IspH bound to 11 . ( c ) Binding of 4-hydroxybutyl diphosphate ( 13 ) to IspH results in formation of an η 1 -alkoxide (or possibly, an alcohol) complex with the apical iron of the [Fe 4 S 4 ] cluster. In addition, one water molecule is evident in the W2 site. Full size image The results presented above all indicate that the 2H + /2e − reductase IspH, which physiologically catalyses the reductive dehydroxylation of HMBPP to form isopentenyl diphosphate and dimethylallyl diphosphate, is promiscuous. The root cause of this promiscuity involves the addition or removal of OH groups at C4 in bound ligands ( Fig. 8 ). The substrate HMBPP ( 1 ) forms a complex with the fourth Fe via O4 and under reducing conditions dehydroxylation ensues ( Fig. 8a ). The alcohol 13 binds to the apical iron via the 4-OH as an alkoxide (or alcohol; Fig. 8b ), but contrary to the situation found with aconitase, no dehydration occurs. The C 3 side chain of the acetylene 4 is too short to interact directly with the oxidised cluster ( Fig. 8c ), but with the C 4 species 5 , a hydroxide (presumably from a cluster-bound water molecule) adds to C4 via anti-Markovnikov addition to form the η 1 -O-enolate 7 , which is subsequently released as the aldehyde 8 ( Fig. 8d ). With a C 5 side chain in 6 , oxygen once again adds at C4, but now, protonation must be at C5 (Markovnikov addition) resulting in the formation of ketone 10 ( Fig. 8e ). The conversion of these IspH substrates is only catalysed by the oxidised form of IspH, no reaction is observed with the reduced protein. These results thus reveal an unexpected side to IspH reactivity, which can be expected to be of importance in inhibitor design and potentially, in chemical synthesis. In addition, these data support the idea that metal–enolate complexes may be involved in acetylene hydratase activity in other systems, as proposed on theoretical grounds [17] . 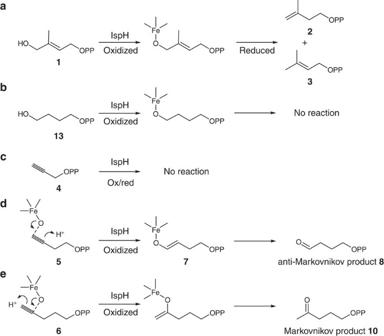Figure 8: Schematic presentation of the diverse reactions catalysed by the [Fe4S4] cluster-containing protein IspH. (a) The unsaturated alcohol1[(E)-4-hydroxy-3-methylbut-2-enyl diphosphate] binds to the cluster and is reductively dehydroxylated to isopentenyl diphosphate (2) and dimethylallyl diphosphate (3). (b) The C4alcohol13binds to oxidised IspH but does not react further. (c) The C3alkyne4is not converted by oxidised or reduced IspH. (d) The C4alkyne5is hydrated at C4 in anti-Markovnikov fashion forming an η1-enolate bound to the apical iron of the [Fe4S4] cluster, resulting in the aldehyde8. (e) The C5alkyne6reacts with oxidised IspH at C4, this time to form the ketone10in a Markovnikov addition. Notably, all reactions involve interactions of the apical iron in the cluster with the oxygen bound to C4 of the ligands. Figure 8: Schematic presentation of the diverse reactions catalysed by the [Fe 4 S 4 ] cluster-containing protein IspH. ( a ) The unsaturated alcohol 1 [( E )-4-hydroxy-3-methylbut-2-enyl diphosphate] binds to the cluster and is reductively dehydroxylated to isopentenyl diphosphate ( 2 ) and dimethylallyl diphosphate ( 3 ). ( b ) The C 4 alcohol 13 binds to oxidised IspH but does not react further. ( c ) The C 3 alkyne 4 is not converted by oxidised or reduced IspH. ( d ) The C 4 alkyne 5 is hydrated at C4 in anti-Markovnikov fashion forming an η 1 -enolate bound to the apical iron of the [Fe 4 S 4 ] cluster, resulting in the aldehyde 8 . ( e ) The C 5 alkyne 6 reacts with oxidised IspH at C4, this time to form the ketone 10 in a Markovnikov addition. Notably, all reactions involve interactions of the apical iron in the cluster with the oxygen bound to C4 of the ligands. Full size image Synthetic protocols All reagents utilized were purchased from Aldrich (Milwaukee, WI). The purity of each compound investigated was confirmed by 1 H and 31 P NMR spectroscopy at 400 MHz or 500 MHz performed on Varian (Palo Alto, CA) Unity spectrometers. Cellulose thin layer chromatography (TLC) plates were visualized by using iodine or a sulphosalicylic acid-ferric chloride stain. The syntheses and characterization of 4 – 6 , 8 , 9 and 11 were described previously [18] , [22] . General procedure for preparation of diphosphates Diphosphates were prepared using modified literature procedures [24] . Typically, 1 mmol of halide or mesylate in a minimum amount of CH 3 CN (0.5 ml) was added drop-wise to a stirred solution of 2.70 g (3.0 mmol) tris(tetra- n -butylammonium)hydrogen diphosphate in CH 3 CN (4 ml) at 0 °C. The reaction mixture was stirred for 2–24 h at room temperature and the solvent was removed under reduced pressure. The residue was dissolved in cation-exchange buffer (49:1 (v/v) 25 mM NH 4 HCO 3 /2-propanol) and slowly passed over 60–100 mequiv Dowex AG50W-X8 (100–200 mesh, ammonium form) cation-exchange resin, pre-equilibrated with volumes of the same buffer. The product was eluted with two column volumes of the same buffer, flash frozen, and lyophilized. The resulting powder was dissolved in 3 ml of 50 mM NH 4 HCO 3 . Nine millilitre of 2-propanol/CH 3 CN (1:1 (v/v)) was added, mixed, centrifuged for 5 min at 2000 r.p.m., and the supernatant was subsequently decanted. This procedure was repeated three times and the supernatants were combined. After solvent removal and lyophilization, followed by flash chromatography on cellulose, a white solid was obtained. Synthesis of compounds 4-Oxobutyl diphosphate 8 and its hydrate 9 were prepared as reported previously for the 3-methyl substituted analogue [22] . 1 H NMR (400 MHz, D 2 O): δ , 9.70. (s, 1H), 5.15-5.05 (br, 1H), 4.00–3.86 (m, 4H), 2.66 ( t , J =6.4 Hz, 2H), 1.98–1.88 (m, 2H), 1.75-1.65 (m, 4H); 31 P NMR(162 MHz, D 2 O): δ , −4.64, −4.78 (two sets dd, J =22 Hz), −8.65, −8.77 (two sets dd, J =22 Hz). Buta-2,3-dienyl diphosphate (12) Buta-2,3-dienyl methane sulphonate (148 mg, 1 mmol) in CH 3 CN (0.5 ml) was treated with 2.7 g (3 mmol) tris(tetra- n -butylammonium)hydrogen diphosphate in CH 3 CN (4 ml). Flash chromatography on a cellulose column (2:1:1 (v/v/v) 2-propanol/CH 3 CN/50 mM NH 4 HCO 3 ) yielded 84 mg (30%) of a white solid. 1 H NMR (400 MHz, D 2 O): δ , 5.26-5.18 (m, 1H), 4.77-4.72 (m, 2H), 4.32-4.25 (m, 2H); 31 P NMR (162 MHz, D 2 O): δ , -9.28 (d, J =20.7 Hz), −10.04 (d, J =20.7 Hz). 13 C NMR (125 MHz, D 2 O): δ , 209.1, 87.7, 76.6, 64.2; high-resolution mass spectrometry (HRMS, ESI) calcd. for C 4 H 9 O 7 P 2 [M+H] + , 230.9824; found 230.9834. 4-Hydroxybutyl diphosphate (13) 4-Chloro-1-butanol (108 mg, 1 mmol) in CH 3 CN (0.5 ml) was treated with 2.7 g (3 mmol) tris(tetra-n-butylammonium)hydrogen diphosphate in CH 3 CN (4 ml). Flash chromatography on a cellulose column (2:1 (v/v) 2-propanol/50 mM NH 4 HCO 3 ) yielded 105 mg (35%) of a white solid. 1 H NMR (400 MHz, D 2 O): δ , 3.79 (dd, J =12.4, 6.0 Hz, 2H), 3.47 (t, J =6.0 Hz, 2H), 1.54-1.43 (m, 4H); 31 P NMR (162 MHz, D 2 O): δ , −9.46 (d, J =21.0 Hz), −9.73 (d, J =21.0 Hz); 13 C NMR (125 MHz, D 2 O): δ , 66.5, 61.6, 27.8, 26.4; HRMS (ESI) calcd. for C 4 H 13 O 8 P 2 [M+H] + , 251.0086; found, 251.0096. Protein purification E. coli IspH for crystallization was prepared as reported previously [9] . Protein for spectroscopic analysis was obtained according to the protocol described below. BL-21 (DE3) cells overexpressing E. coli IspH (encoded in plasmid pASK-IBA3 + ) and Isc proteins (encoded in plasmid pDB1282) were grown in Luria-Bertani media supplemented with 100 mg l –1 ampicillin and 50 mg l –1 kanamycin at 37 °C, until the OD 600 reached 0.3. Cells were then induced with 0.5 g l –1 arabinose to initiate overexpression of the Isc proteins. Cysteine (1 mM) and FeCl 3 (0.1 mM) were supplemented, and cells were grown until the OD 600 reached 0.6. At this point, 400 μg l –1 anhydro-tetracycline was added to induce overexpression of IspH. Cells were grown at 25 °C for 16 h, harvested by centrifugation and kept at −80 °C until use. All purification steps were carried out in a Coy Vinyl Anaerobic Chamber (Coy Laboratories, Grass Lake, MI) with an oxygen level <2 p.p.m., and all buffers were degassed by using a Schlenk line. Cell pellets were re-suspended in 100 mM Tris/HCl, 150 mM NaCl buffer (pH 8.0). Lysozyme, Benzonase nuclease (EMD Chemicals, San Diego, CA) and phenylmethanesulfonyl fluoride were added, and the mixture was stirred for 1 h at 10 °C followed by sonication (Fisher Scientific Sonic Dismembrator, Model 500) with four pulses, each 7 s duration, at 35% power. The cell lysate was centrifuged at 11,000 r.p.m. at 10 °C for 30 min. The supernatant was purified by using Strep-tactin chromatography [25] . Fractions having a brown colour were collected and desalted in pH 8.0 buffer containing 100 mM Tris/HCl and 150 mM NaCl. 57 Fe-enriched IspH was prepared following the same procedures as for natural-abundance IspH, described above, except that 57 Fe metal dissolved in HCl was added to the Luria-Bertani media to a final concentration of 80 μM. Spectroscopy Mößbauer spectra were recorded on a constant acceleration spectrometer (Knox College) at 77 K with a 500G magnetic field perpendicular to the γ-ray. NMR spectra were collected on a 500 MHz Varian Unity spectrometer and ESI–MS spectroscopy was performed on a Waters Quattro II mass spectrometer. Crystallization Co-crystallization of IspH and the inhibitors was performed under anaerobic conditions in a Coy Vinyl Anaerobic Chamber (Coy Laboratories, Grass Lake, MI) with an N 2 /H 2 (95%/5%) atmosphere. All buffers were refluxed for 20 min and were stored under argon. A 100 mM aqueous solution of each inhibitor was prepared with degassed water and stored under anaerobic conditions at −80 °C. A protein solution with a concentration of 18.3 mg ml –1 was incubated with 1 mM inhibitor before crystallization. Dark brown crystals were obtained by using the sitting drop vapour diffusion method at 20 °C with 100 mM BisTris/HCl, pH 6.5, 200 mM ammonium sulphate and 25% polyethylene glycol 3350 as precipitant. Crystals were soaked with cryo-protectant solution (50% aqueous polyethylene glycol 400) for 1 min, mounted on loops and flash cooled in a stream of nitrogen gas at 100 K (Oxford Cryo Systems). Data collection and structure determination Native data sets were collected at 1.0 Å and 100 K using synchrotron radiation at the X06SA-beamline at the Swiss Light Source, Villigen, Switzerland and at the ID29-beamline at the European Synchrotron Radiation Facility, Grenoble, France. The phase problem was solved by molecular replacement using the coordinates of E. coli IspH bound to the substrate HMBPP (PDB [26] ID: 3KE8) as the starting model [9] . Data were processed using the program package XDS [27] . The anisotropy of diffraction was corrected using TLS refinement [28] . Model building and refinement were performed with Coot [29] and Refmac [30] . Figures were prepared using PyMOL [31] and Ramachandran plots were calculated with PROCHECK [32] . Ramachandran statistics for the refined structures are 98.7/1.3/0.0 (Crystal 1 IspH: 4 ), 98.8/1.2/0.0 (Crystal 2 IspH: 7 ), 98.4/1.6/0.0 (Crystal 3 IspH: 8 ), 99.0/1.0/0.0 (Crystal 4 IspH: 10 ), 99.0/1.0/0.0 (Crystal 5 IspH: 11 ), 98.9/1.1/0.0 (Crystal 6 IspH: 12 ) and 99.0/1.0/0.0 (Crystal 7 IspH: 13 ). For more details see Supplementary tables S1 and S2 . Accession codes: Coordinates and structure factors for IspH in complex with the ligands 4 , 7 , 8 , 10 , 11 , 12 and 13 have been deposited in the Protein Data Bank under accession codes 3URK , 3UTC , 3UWM , 3UTD , 3UV3 , 3UV7 and 3UV6 , respectively. How to cite this article: Span, I. et al . Discovery of acetylene hydratase activity of the iron-sulphur protein IspH. Nat. Commun. 3:1042 doi: 10.1038/ncomms2052 (2012).